Lateralized enhancement of auditory cortex activity and increased sensitivity to self-generated sounds Performing actions with auditory consequences modulates the response in auditory cortex to otherwise identical stimuli passively heard. Such modulation has been suggested to occur through a corollary discharge sent from the motor cortex during voluntary actions. However, the relationship between the effector used to generate the sound, type of modulation and changes in perceptual sensitivity are unclear. Here we use functional magnetic resonance imaging on healthy subjects and demonstrate bilateral enhancement in the auditory cortex to self-generated versus externally generated sounds. Furthermore, we find that this enhancement is stronger when the sound-producing hand is contralateral to the auditory cortex. At the behavioural level, binaural hearing thresholds are lower for self-generated sounds and monaural thresholds are lower for sounds triggered by the hand ipsilateral to the stimulated ear. Together with functional connectivity analysis, our results suggest that a corollary discharge sent from active motor cortex enhances activity in the auditory cortex and increases perceptual sensitivity in a lateralized manner. Performing an action, such as pressing a button to ring the doorbell, entails sensory consequences in different sensory modalities. Identical sensory consequences can arise when similar actions are performed by others (for example, the auditory consequences in the case someone else pressed the button to ring the bell). A pure sensory system should in principle respond to both types of sensory consequences in the same manner. However, research over the past few decades has demonstrated that at the behavioural level, self-generated and externally generated sensory consequences are perceived differently, and at the physiological level they evoke different neural responses in sensory regions [1] , [2] . This differential response is believed to occur through a ‘corollary discharge’ [3] , or ‘efference copy’ [4] that is sent by the motor cortex, as part of an internal forward model [5] to sensory areas before self-generated voluntary action. The postulated model for sensory processing of self-generated stimuli implies that during voluntary movement, the motor commands are sent to the executing effectors and, in parallel, a copy is sent to the relevant sensory cortex in which action–consequences of the voluntary action are expected. This copy can inhibit, excite or otherwise modulate the activity in the sensory cortex [4] and is considered to be an essential component of a forward model that is involved in online correction of movements based on sensory feedforward–feedback ‘errors’ [5] . The role of efference copies has been examined at many physiological levels. Intracellular recordings from auditory afferent neurons of crickets showed an inhibited firing pattern during self-generated acoustic stimulation—an inhibition that is believed to prevent desensitization of auditory pathways. Such inhibition can consequently allow the cricket to respond and maintain sensitivity to external sources of acoustic stimulation such as singing of other crickets [6] . In primates, several studies examined neural activity in the auditory cortex during self-initiated vocalizations. Eliades and Wang [7] have shown that the majority of neurons in the auditory cortex reduce their firing rates starting ~200 ms before the onset of animal vocalization, while another subset of neurons increases their firing rate at the onset of vocalization. It has been suggested that the neurons with reduced firing rates are modulated by the preceding motor commands (efference copies) and the neurons showing increased firing rates respond to the re-afferent auditory feedback. In humans, responses to self-produced versus externally produced sensory stimuli have been studied both at the behavioural and physiological levels. At the behavioural level, self-produced tactile stimulation is perceived as less ticklish compared with identical tactile stimulation produced by an external source [8] . In the auditory modality, when subjects compare the loudness of two identical sounds—one produced by actively pressing a button and the other perceived passively—the sound in the active condition is reported as being less loud [9] . In contrast, proprioceptive sensation has been shown to be enhanced during self-generated movements, with fewer errors made regarding spatial hand position when hand displacement is self-generated compared with passive displacement [10] . At the physiological level, the phenomenon of sensory modulation in humans has been explored using various techniques. In magnetoencephalography and electroencephalography studies using speech or tones, the evoked response in frontocentral regions is reduced in active compared with passive conditions [11] , [12] , [13] , [14] . However, using visual feedback one study reports enhanced evoked responses in occipital regions during active compared with passive conditions [15] . Using transcranial magnetic stimulation (TMS), it has been shown that even during motor preparation (that is, before the actual motor act) sensitivity to sensory stimuli is already reduced [16] . Invasive studies in patients, using electrocorticography show mostly suppressed responses in superior temporal gyrus (STG) to self-vocalization versus passive listening to similar speech sounds [17] , [18] . Functional imaging data on the other hand are more mixed, with some studies showing enhancement, others showing attenuation, and yet others showing both phenomena in different brain regions within the same subjects. Using ischaemic nerve block it has been shown that during voluntary movement, functional magnetic resonance imaging (fMRI) signal in primary somatosensory cortex (S1) is enhanced (even in the lack of sensory feedback) and functional connectivity with pre-motor cortex is increased, suggesting an enhancing effect of a motor efference copy [19] . Similarly, using positron-emission tomography it has been shown that increases in speech production rate result in increased cerebral blood flow in auditory cortices even when auditory feedback was blocked by white noise that was kept constant across rates [20] . Other studies report enhancement of the fMRI signal in S1 during perception of self-generated tactile stimuli compared with similar stimuli externally generated [21] , [22] . Finally, the fMRI signal in the auditory cortex during active speaking (relative to passive listening) has been shown to be attenuated in STG but enhanced in superior temporal sulcus of the same subjects [23] . While some studies report reduced neural activity (at the physiological level) or reduced sensitivity (at the behavioural level) to self-generated action–consequences, other studies show enhancement. Given the relative paucity of fMRI studies examining this issue at the whole-brain level, the network of brain regions involved in sensory modulation during voluntary movement, the type of modulation they undergo (enhancement or attenuation) and their relation with behaviour is not clear. Although the motor system is highly lateralized (with a predominance of each hemisphere controlling the contralateral side) and anatomical evidence [24] , [25] suggesting stronger connectivity between motor and auditory cortices residing in the same hemisphere, it is unclear whether such modulations depend on the identity of the performing hand. To this end, we used fMRI to examine sensory modulation while subjects heard identical sounds either during active keyboard playing or passive listening. We further examined whether this modulation depends on the identity of the sound-producing hand. Our results show that sensory attenuation is mostly found in frontal regions such as the superior and middle frontal gyri (SFG and MFG) bilaterally. In contrast, activity in auditory cortices (bilateral STG) is enhanced during the active condition. Furthermore, this enhancement is stronger when the performing hand is contralateral to the auditory cortex. This lateralized enhanced response in the auditory cortex is further supported at the behavioural level as manifested by lower hearing thresholds to sounds evoked by the hand ipsilateral to the stimulated ear. fMRI study We performed whole-brain fMRI scans on healthy subjects while they played or heard short unimanual piano melodies. Under the active condition, subjects played a 7-note melody with either their right or left hand on an MR-compatible digital piano keyboard while online auditory feedback was provided through earphones. The auditory feedback in this condition was recorded and subsequently replayed to the subjects in the passive condition, thus maintaining identical sensory stimulation across the two conditions ( Fig. 1 ). 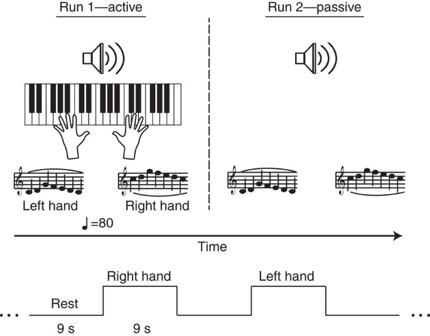Figure 1: Experimental design. The experiment consisted of two runs arranged in a block design. In the first run, subjects played a short musical sequence on a digital MRI-compatible piano keyboard with either their right or left hands while online auditory feedback was provided through earphones (active condition). Subjects were given 9 s to play the sequence after a visual cue indicating which hand to use. In the second run, subjects passively listened to the playback of their own performance recorded during the first run (passive condition). Figure 1: Experimental design. The experiment consisted of two runs arranged in a block design. In the first run, subjects played a short musical sequence on a digital MRI-compatible piano keyboard with either their right or left hands while online auditory feedback was provided through earphones (active condition). Subjects were given 9 s to play the sequence after a visual cue indicating which hand to use. In the second run, subjects passively listened to the playback of their own performance recorded during the first run (passive condition). Full size image On the basis of previous studies reporting mostly attenuated auditory responses during vocalization or perception of self-generated sounds, we first examined which brain regions manifest attenuated auditory responses under the active versus passive condition. Using a contrast of passive>active condition in each subject, we found significant voxels (corrected for false discovery rate q(FDR)<0.05) in the MFG and the medial part of SFG bilaterally. 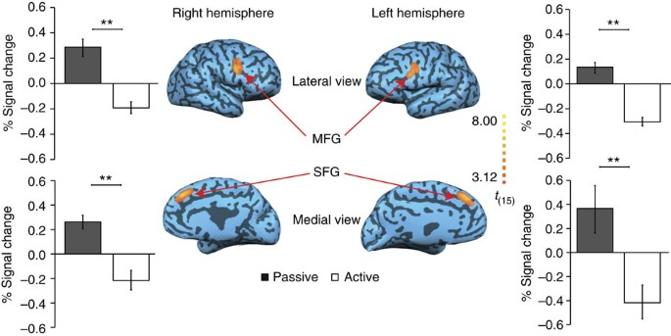Figure 2: Sensory attenuation in the frontal lobe during active playing. Random effect multistudy map (n=16; corrected for q(FDR)<0.05) showing regions in MFG (lateral view) and SFG (medial view) with stronger fMRI signal in the passive compared with active conditions. Bar graphs represent the average±s.e.m. fMRI signal across individual subjects in the corresponding regions (two-tailed pairedt-test, **P<0.001). Mean±s.e.m. Talairach coordinates in right MFG (n=11):x=37.6±2.2,y=4.8±2.7,z=43.8±3.1; left MFG (n=13):x=−41.7±2.6,y=9.1±2.6,z=42.3±2.4; right SFG (n=10):x=3.8±0.6,y=27.4±3.7,z=49.2±2.2; left SFG (n=12):x=−5.6±1.1,y=30.1.4±4.4,z=42.5±2.8. Figure 2 displays the multisubject map ( n =16) obtained with this contrast. Figure 2: Sensory attenuation in the frontal lobe during active playing. Random effect multistudy map ( n =16; corrected for q(FDR)<0.05) showing regions in MFG (lateral view) and SFG (medial view) with stronger fMRI signal in the passive compared with active conditions. Bar graphs represent the average±s.e.m. fMRI signal across individual subjects in the corresponding regions (two-tailed paired t -test, ** P <0.001). Mean±s.e.m. Talairach coordinates in right MFG ( n =11): x =37.6±2.2, y =4.8±2.7, z =43.8±3.1; left MFG ( n =13): x =−41.7±2.6, y =9.1±2.6, z =42.3±2.4; right SFG ( n =10): x =3.8±0.6, y =27.4±3.7, z =49.2±2.2; left SFG ( n =12): x =−5.6±1.1, y =30.1.4±4.4, z =42.5±2.8. Full size image Interestingly, the contrast of passive>active conditions yielded no significant voxels in auditory cortex. In order to directly examine potential modulation effects of the active condition in the auditory cortex, we first defined for each subject auditory regions of interest (ROIs) using a contrast of passive>rest in an independent localizer experiment (see Methods and Fig. 3a for multisubject map). ROI selection was restricted to the middle part of the STG in both hemispheres for subsequent analysis (mean±s.e.m. Talairach coordinates across subjects in right STG: x =56.4±1.4, y =−23.5±1.4, z =7.4±0.8; left STG: x =−59.7±1.0, y =−26.7±1.3, z =6.3±1.3). 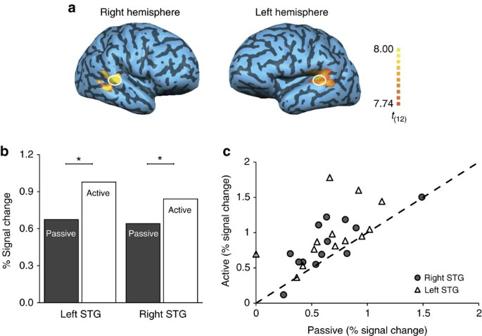Figure 3: Sensory enhancement in the auditory cortex during active playing. (a) Random effect multistudy map (n=13; corrected for q(FDR)<0.05) using a contrast of passive condition>rest from the auditory localizer runs. White circles show the average auditory ROIs across subjects in Middle Superior Temporal Gyri. (b) The mean response across subjects (% signal change) in the main experiment was greater during active compared with passive conditions both in left (n=13) and right (n=13) STG (two-tailed pairedt-test; *P<0.05). (c) Individual subject responses in left and right STG during active and passive conditions. The dashed line represents equal signal strength across the two conditions. Note that in most of the subjects, activation in STG during the active condition was greater than during the passive condition. Figure 3: Sensory enhancement in the auditory cortex during active playing. ( a ) Random effect multistudy map ( n =13; corrected for q(FDR)<0.05) using a contrast of passive condition>rest from the auditory localizer runs. White circles show the average auditory ROIs across subjects in Middle Superior Temporal Gyri. ( b ) The mean response across subjects (% signal change) in the main experiment was greater during active compared with passive conditions both in left ( n =13) and right ( n =13) STG (two-tailed paired t -test; * P <0.05). ( c ) Individual subject responses in left and right STG during active and passive conditions. The dashed line represents equal signal strength across the two conditions. Note that in most of the subjects, activation in STG during the active condition was greater than during the passive condition. Full size image In each subject we compared the evoked signal under the active and passive conditions within the ROI and found that the fMRI signal was enhanced during the active condition both in right and left STG (mean±s.e.m. : right STG: 0.83±0.1% active condition, 0.64±0.08% passive condition; n =13, two-tailed paired t-test , t (12) =3.11, P =0.009; left STG: 0.97±0.11% active condition, 0.67±0.08% passive condition; n =13, t (12) =3.2, P =0.006; see group average and individual subjects data in Fig. 3 ). In order to use identical auditory stimuli across the active and passive conditions, self-generated sounds in the active condition were recorded and replayed during the passive condition. This introduced an inherent order effect in the experimental design, which is unavoidable and could potentially explain the enhanced fMRI signal under the active condition. In order to rule this out, 11 of the subjects also passively listened to a novel 7-note melody in two consecutive runs (that is, two passive runs). We examined whether there was a decrease in signal strength in the second run compared with the first (similar to what we observed between the active and passive runs). No significant decrease in signal strength was evident in the right (mean±s.e.m. : 0.89±0.1% first run; 0.92±0.09% second run, n =11, one-tailed paired t-test , t (10) =0.41, P =0.43) and left (1.11±0.16% first run; 1.16±0.16% second run, n =11, t (10) =0.64, P =0.24) STG ROIs. This was also true after collapsing the data across both right and left STGs ( n =22, t (21) =1.25, P =0.22; see Supplementary Fig. 1 ). Thus, fMRI signal enhancement in STG reported in the main experiment is most likely not due to condition order. It might be argued that our 7-note long musical sequences required high levels of attention, possibly explaining the difference between the active and passive conditions. We note that the subjects trained on these sequences for 30 min the day before the scan, and again for 10 min right before the scan. Indeed, their performance level during the scan was at ceiling (mean±s.e.m. % correct button presses across subjects: 95±1.5% at an average rate of 1.6 notes per second), suggesting that the motor sequences were well learned. Although performance levels were high, it is still possible that performing musical sequences requires higher levels of attention during the active compared with passive conditions. In order to examine this possibility, we collected fMRI data from 11 additional subjects who performed the active/passive conditions, using a simpler motor task that does not require training. During the active conditions, subjects triggered short 1 kHz tones with a simple button press using their right index finger at a rate of 1 Hz. During the passive condition, they passively listened to an identical replay of the tones generated in the active condition (see Methods). First, we performed a whole-brain contrast of passive>active as in the main experiment using melodies. We found activations in bilateral MFG and right SFG ( Supplementary Fig. 2 ). Next, we defined auditory ROIs in STG (see Methods). In these ROIs we found that fMRI signal was significantly larger during the active compared with the passive condition (mean±s.e.m. collapsed across right/left STG: active condition: 0.72±0.03%, passive condition: 0.52±0.02%; n =22, two-tailed paired t-test , t (21) =2.05, P =0.02; Supplementary Fig. 3 ). The enhancement effects in STG ROIs using 1 kHz tones or melodies were not significantly different ( n 1 =22, n 2 =26, two-tailed unpaired t-test , t (46) =0.51, P =0.61). Taken together, the activity patterns in frontal and auditory regions using tones are in agreement with the results using musical sequences and suggest that the enhancement effect in the auditory cortex does not depend on differences in attention and performance levels. Next, we examined whether the enhancement observed in STG during the active condition of the main experiment depends on the identity of the performing hand. We found that the fMRI signal in left STG was higher when subjects played the 7-note melodies with their right hand compared with when they played with their left hand (mean±s.e.m. : right hand: 1.06±0.12%; left hand: 0.89±0.1%; n =13; two-tailed paired t-test , t (12) =2.9; P =0.01). The opposite was true in right STG—activity was higher when subjects played with their left hand compared with when they played with their right hand (left hand: 0.91±0.12%; right hand: 0.75±0.08%; n =13; t (12) =2.6; P =0.02; see group average and individual subject data in Fig. 4 ). 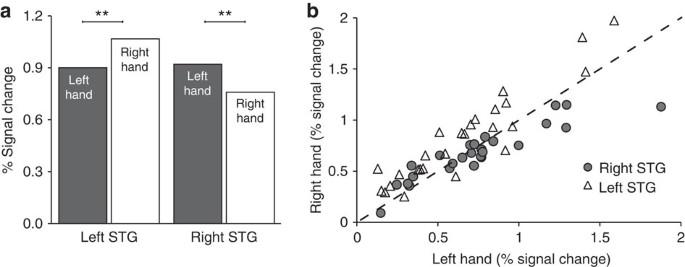Figure 4: Hand identity modulates auditory responses in a lateralized manner. (a) The mean response across subjects (% signal change) in left STG was greater when subjects played the musical sequence with their right compared with their left hands (n=13; two-tailed pairedt-test, **P<0.01). Symmetrically, response in right STG was greater when the subjects played the musical sequence with their left compared with their right hands (n=13; **P<0.01). (b) Individual subject responses in right and left STG as a function of executing hand. The dashed line represents equal signal strength across the two conditions. Note the separation between right and left STG (see alsoSupplementary Fig. 4). Figure 4: Hand identity modulates auditory responses in a lateralized manner. ( a ) The mean response across subjects (% signal change) in left STG was greater when subjects played the musical sequence with their right compared with their left hands ( n =13; two-tailed paired t -test, ** P <0.01). Symmetrically, response in right STG was greater when the subjects played the musical sequence with their left compared with their right hands ( n =13; ** P <0.01). ( b ) Individual subject responses in right and left STG as a function of executing hand. The dashed line represents equal signal strength across the two conditions. Note the separation between right and left STG (see also Supplementary Fig. 4 ). Full size image The Talairach coordinates of our STG ROIs lie close to the secondary somatosensory area (SII), located at the upper bank of the Lateral Sulcus [26] . In order to exclude possible contamination of our STG ROI by voxels from SII, we conducted a control experiment (similar design as the main experiment using melodies) in which our subjects also performed a visual-motor task during which they typed 7-digit numbers with their right (‘3-4-1-3-4-5-1’) or left (‘1-5-4-3-1-4-3’) hands by pressing the digital piano keys and receiving visual feedback of the typed numbers (1 corresponding to the thumb and 5 to the little finger). Importantly, this task involved similar tactile input as the main experiment but had no auditory component. We found that the signal modulation in our STG ROI was not significantly different than zero during this task in left and right STG ( n =13, two-tailed paired t-test , left STG: t (12) =1.6, P =0.12; right STG: t (12) =1.96, P =0.07). Furthermore, we found no laterality effect neither in right (mean±s.e.m. : 0.09±0.05% right hand; 0.12±0.05% left hand, n =13, two-tailed paired t-test , t (12) =0.48, P =0.73) nor left (0.14±0.09% right hand; 0.16±0.19% left hand, n =13, t (12) =0.42, P =0.83) STGs. Group average and individual subject data are provided in Supplementary Fig. 4 . Therefore, the lateralized enhancement in STG reported in the main experiment seems to be better explained by the audio-motor coupling between the hand and sound it produces rather than by a global hemispheric effect or contamination of our STG ROI by voxels in contralateral SII responding to tactile feedback from the playing hand. We also used the fMRI data to examine functional connectivity between the motor cortex and all other regions of the brain during left and right hand melody playing. To that end, we performed psychophysiological interaction (PPI) analysis using left and right primary motor cortex as seed regions (see Methods for details). We found that during right hand playing, activity in the left motor cortex was most strongly connected with the left STG (across all brain regions). Similarly, during left hand playing, activity in the right motor cortex was most strongly connected with the right STG. Thus, the active motor cortex had highest functional connectivity with the auditory cortex residing in the same hemisphere ( Fig. 5 ). 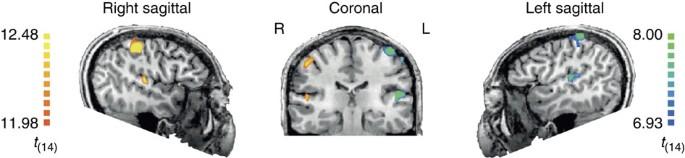Figure 5: Functional connectivity between ipsilateral motor and auditory cortices. Random effect multistudy map (n=15) showing the most significant voxels (corrected for q(FDR)<0.005) in left hand>right hand contrast of PPI analysis (see Methods). Using the right motor cortex as seed region, the right auditory cortex had the strongest functional connectivity, over all other brain regions, during left (compared with right) hand playing (red). Symmetrically, using the left motor cortex as seed region, the left auditory cortex had the strongest functional connectivity during right (compared with left) hand playing (blue). Coronal view: R, right hemisphere; L, left hemisphere. Figure 5: Functional connectivity between ipsilateral motor and auditory cortices. Random effect multistudy map ( n =15) showing the most significant voxels (corrected for q(FDR)<0.005) in left hand>right hand contrast of PPI analysis (see Methods). Using the right motor cortex as seed region, the right auditory cortex had the strongest functional connectivity, over all other brain regions, during left (compared with right) hand playing (red). Symmetrically, using the left motor cortex as seed region, the left auditory cortex had the strongest functional connectivity during right (compared with left) hand playing (blue). Coronal view: R, right hemisphere; L, left hemisphere. Full size image In addition, we examined whether during the active condition, the identity of the playing hand (right/left) could be determined based on the patterns of fMRI signal in various brain regions in individual trials. To that end, the fMRI signal from multiple voxels was used as input to a linear classification algorithm (see Methods). The classification performance across subjects was significantly above chance based on activity patterns of voxels in right and left STG ROIs (mean±s.e.m. 71.25±4.42% n =12; t (11) =5.24, P <10 −3 ) but not based on voxels in SFG (55.1±5.45% n =10; ns) or MFG ROIs (56.18±5.28% n =11; ns; Supplementary Fig. 5 ). For reference, the mean classification performance of hand identity from the primary motor cortex (defined by a contrast of right hand>left hand) was 97.7±1.0%. Behavioural study Since fMRI activity in the auditory cortex has been previously shown to correlate with perceived loudness of auditory stimuli [27] , in an additional set of behavioural experiments we examined whether the fMRI results in our study also have a behavioural correlate of increased hearing sensitivity. First, we performed an experiment in which we assessed binaural hearing thresholds to a 1-kHz pure-tone in 16 subjects during active and passive conditions (see Methods for details). In agreement with the fMRI data, thresholds in the active condition were significantly lower compared with thresholds in the passive condition (mean±s.e.m. : −3.45±1.19 dBHL active condition; −2.31±1.16 dBHL passive condition; n =16, one-tailed paired t-test , t (15) =3.01, P =8 × 10 −3 ; see group average and individual subject data in Fig. 6 ). 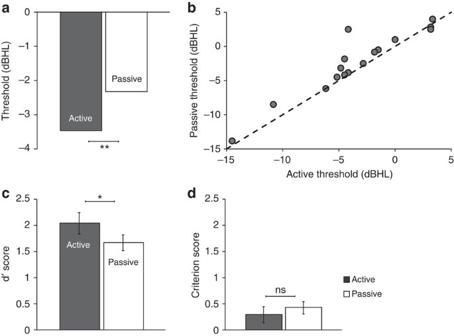Figure 6: Binaural hearing thresholds. (a) The mean hearing threshold to a 1-kHz pure tone in the active condition was lower compared with the passive condition (n=16; one-tailed pairedt-test; **P<0.01). (b) Hearing thresholds in active and passive conditions for individual subjects. The dashed line represents equal detection threshold across the two conditions. Note that most subjects had higher thresholds in the passive condition. (c) Mean (±s.e.m.) d′ score across subjects—mean d′ score was higher in active compared with passive conditions (n=10; one-tailed pairedt-test; *P<0.05) indicating increased sensitivity in this condition. (d) The mean (±s.e.m.) criterion score across subjects—the mean criterion score did not significantly differ across active and passive conditions (n=10; two-tailed pairedt-test;P=0.08). Figure 6: Binaural hearing thresholds. ( a ) The mean hearing threshold to a 1-kHz pure tone in the active condition was lower compared with the passive condition ( n =16; one-tailed paired t -test; ** P <0.01). ( b ) Hearing thresholds in active and passive conditions for individual subjects. The dashed line represents equal detection threshold across the two conditions. Note that most subjects had higher thresholds in the passive condition. ( c ) Mean (±s.e.m.) d′ score across subjects—mean d′ score was higher in active compared with passive conditions ( n =10; one-tailed paired t -test; * P <0.05) indicating increased sensitivity in this condition. ( d ) The mean (±s.e.m.) criterion score across subjects—the mean criterion score did not significantly differ across active and passive conditions ( n =10; two-tailed paired t -test; P =0.08). Full size image The reduced threshold we observed in the active compared with the passive conditions could, in principle, be the result of a change in subject’s criterion rather than a true reduction in hearing sensitivity. Thus, a change in probability of saying ‘yes’ (tone detected) in the active condition might result in reduced threshold while true hearing sensitivity has not changed. In order to examine this issue, we utilized the hit and false-alarm rates in an auditory detection task to assess sensitivity (d′) and criterion (c) measures for the active and passive conditions in 10 subjects (see Methods for details). D-prime, which is a measure of sensitivity independent of criterion, was higher for the active compared with the passive condition supporting a true increase in sensitivity (mean±s.e.m. d′: 2.03±0.2 active condition, 1.66±0.15 passive condition; n =10; one-tailed paired t-test , t (9) =1.97, P =0.04; Fig. 6c ). Criterion measure was slightly higher in the passive compared with the active condition, although this difference failed to reach statistical significance (mean±s.e.m. c: 0.42±0.11 active condition, 0.29±0.15 passive condition; two-tailed paired t-test , t (9) =1.9, P =0.08; Fig. 6d ). The higher d′ in the active condition was mostly due to increase in hit rate (mean±s.e.m. : 0.75±0.03% active condition, 0.65±0.03% passive condition ; two-tailed paired t-test , t (9) =2.9, P =0.02) and no significant change in false-alarm rate (mean±s.e.m. : 0.14±0.05% active condition, 0.13±0.04% passive condition; two-tailed paired t-test , t (9) =0.41, P =0.69). Taken together, these results demonstrate that the reduced thresholds in the active condition represent a true increase in sensitivity and are unlikely to be explained solely by a mere change in criterion. Given that monaural stimulation evokes activity biased to the contralateral hemisphere [28] , we examined the relationship between identity of the active hand (right or left) and monaural hearing thresholds in each ear in 13 subjects. Subjects generated sounds by pressing a key with either their right or left hand (see Methods for details). Compatible with the laterality effect we observed in the fMRI data, detection thresholds were lower when the active hand was ipsilateral compared with contralateral to the stimulated ear (mean±s.e.m. : −1.17±0.75 dBHL ipsilateral; −0.25±0.75 dBHL contralateral; n =22 ears; one-tailed paired t-test , t (21) =2.18, P =0.02). In other words, when motor activity and evoked auditory response are in the same hemisphere, detection threshold is lower. For example, detection threshold in the right ear was lower when the sound was produced by right-hand button presses compared with left-hand button presses (and vice versa in the left ear). Group average and individual subject data are shown in Fig. 7 . Seven subjects (out of 13) performed the monaural threshold evaluation task while the executing hand was in the opposite hemifield (that is, right hand key presses were performed in the left hemifield and left hand key presses were performed in the right hemifield). Monaural threshold in the ear ipsilateral to the performing hand (for example, right ear and right hand) was still lower compared with the threshold obtained while using the contralateral hand (for example, right ear left hand; mean±s.e.m. : −2.4±1.44 dB HL ipsilateral hand; −1.13±1.41 dB HL contralateral hand; n =11 ears, one-tailed paired t-test , t (10) =2.16, P =0.028). These results suggest that the monaural threshold advantage to ipsilateral hand does not depend on congruency in spatial field but rather on congruency between the laterality of active hand and stimulated ear. 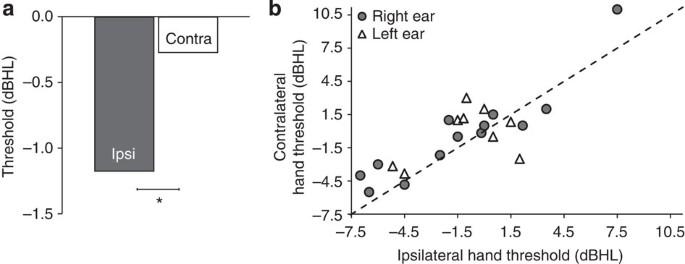Figure 7: Monaural hearing thresholds. (a) Mean hearing threshold was lower when the hand used to trigger the sound was ipsi—compared with contralateral to the stimulated ear (n=22; one-tailed pairedt-test; *P<0.05). (b) Thresholds in ipsi- and contralateral conditions (all ears). The dashed line represents equal detection threshold across the two conditions. Note that in most ears, thresholds were lower when the ipsilateral hand was used to trigger the sound. Figure 7: Monaural hearing thresholds. ( a ) Mean hearing threshold was lower when the hand used to trigger the sound was ipsi—compared with contralateral to the stimulated ear ( n =22; one-tailed paired t -test; * P <0.05). ( b ) Thresholds in ipsi- and contralateral conditions (all ears). The dashed line represents equal detection threshold across the two conditions. Note that in most ears, thresholds were lower when the ipsilateral hand was used to trigger the sound. Full size image The aims of the current study were to examine how performing a voluntary action modulates neural activity during perception, where in the brain these modulations take place, and what is the role of performing hand identity (left versus right) in such modulation. We further set out to examine the correspondence between neural modulation (as assessed using fMRI) and behavioural hearing thresholds. We demonstrated that the fMRI activity in frontal regions such as the MFG and SFG is attenuated under active versus passive conditions. In contrast, activity in the auditory cortex (bilateral STG) during active sound generation is enhanced compared with passive listening to identical sounds. This enhancement was sensitive to the identity of the sound-generating hand such that both in right and left STG we found stronger signal enhancement when the sound-generating hand was on the contralateral side. We also assessed whether these patterns of fMRI activity have a behavioural correlate and found lower binaural hearing thresholds for self-generated versus externally generated sounds. Finally, we also found that monaural hearing thresholds were lower when the sound-generating hand was ipsilateral to the stimulated ear. Anatomical evidence implies stronger connectivity of the auditory cortex with the contralateral ear [29] . In agreement, functional studies using monaural stimulation show stronger activity in the auditory cortex contralateral to the stimulated ear [28] . Therefore, it might support the notion that sounds delivered to one ear are predominantly processed in the contralateral hemisphere. Given that our fMRI results show enhanced activity in STG contralateral to the sound-triggering hand, and that activity in STG has been shown to correlate with perceived loudness [27] , we looked for differences in monaural hearing thresholds for stimuli triggered by the different hands. Right ear stimulation evokes activity in the auditory cortex which is biased to the left hemisphere, and our fMRI results indicate stronger fMRI signal in left STG during playing with the right versus the left hand. Therefore, we predicted that during right ear stimulation, sounds produced by the right hand will result in lower hearing thresholds compared with sounds produced by the left hand (and vice versa for left ear stimulation). Indeed, these predictions were borne out in our behavioural results. Attention has been demonstrated to increase activity in the auditory cortex [30] , [31] . Therefore, it might be argued that increased allocation of attention resources during active playing provides an alternative account to the enhanced fMRI signal in this condition compared with passive listening. While this explanation cannot be completely ruled out, we believe it is unlikely to explain our results. First, the signal enhancement we observed when subjects generated a sequence of tones (comprising a melody) using multiple fingers in a serial manner was also observed when a single sound was repeatedly produced using one finger. This condition is relatively low in attention demand. Second, we employed an oddball detection task in the passive condition that forced the subjects to attend to the stimuli. Third, our main results indicate differential enhancement across hemispheres that depends on identity of the executing hand. This fMRI laterality effect is also in agreement with our behavioural (monaural) results, which held true regardless of the spatial location of the performing hand (left or right hemispace). Taken together, it seems that active sound generation, and moreover hand identity, is a more plausible explanation driving the increased fMRI signal and reduced hearing thresholds. Reduced fMRI signal to repeated stimuli has been demonstrated in various modalities including auditory [32] . Since in our design the passive condition was always a repeat of the active condition, this inherent order could potentially provide an alternative account for the lower signal under the passive condition. Examining this issue using two consecutive passive listening conditions, we did not find reduced signal in the second repeat. Therefore, suppression due to repeated presentation of identical sounds is unlikely to be the source of our effects. A body of literature suggests attenuated neural and behavioural responses in active versus passive conditions, although recent studies have also demonstrated the opposite effect [15] , [21] , [33] , [34] , [35] , suggesting the existence of different modulation types in different brain regions. Many human fMRI and electrocorticography studies reporting attenuation have compared speech production with passive listening to speech sounds [17] , [18] . While the appeal of using speech as a natural stimulus is clear, it nonetheless introduces difficulties in equating the physical attributes of the sound between the passive and active conditions. This is due to sound propagating through air and bone conduction and the contraction of the stapedius muscle during self-vocalization. The contraction of the stapedius muscle (that is, acoustic reflex) during overt speech, results in decreased compliance (stiffening) of the middle ear system and attenuation of self-generated vocal sounds. Interestingly, the stapedius muscle has been shown to contract up to 150 ms before speech onset [36] . In our design, we avoided these issues by using digital sounds (musical or 1 kHz tones) in order to deliver auditory stimuli with identical physical attributes across active/passive conditions. Although the fMRI BOLD signal in auditory cortex has been shown to correlate with modulations in population neural firing rate [37] , we note that it does not provide adequate temporal resolution to determine whether the modulations we report reflect early or late cortical responses. Behavioural studies showing sensory attenuation have used tasks in which subjects generate a sound in the active condition and report perceived sound loudness relative to an externally generated reference sound (for example, refs 9 , 38 ). In addition to auditory networks, these tasks engage cognitive networks such as memory and decision making. In the current study, we tried to avoid this by using a simple detection task to assess hearing thresholds. It is possible that different tasks engage neural mechanisms that are modulated differently by voluntary actions. Our functional connectivity analysis supports the notion that primary motor cortex takes part in the modulation observed in the auditory cortex during voluntary actions. Using primary motor cortex as seed region, functional connectivity during our tasks was strongest with the auditory cortex residing in the same hemisphere. This is in agreement with anatomical evidence indicating stronger interhemispheric connections between both rostral and caudal parts of STG and frontal, pre-motor and primary motor cortices [24] , [25] . Functional mapping using electrical stimulation of auditory regions in humans (such as the posterior–lateral superior temporal cortex) has been shown to evoke activity in ipsilateral frontal regions such as the ventrolateral pre-frontal cortex further supporting the functional connections between auditory and motor regions [39] . Interestingly, pre-motor regions have been shown to contain mirror neurons—nerve cells that respond during execution and passive observation of actions [40] . More relevant here is the discovery of audio-motor mirror neurons in these regions—cells involved in the execution of actions that also respond during passive listening to the sounds evoked by such actions [41] , [42] . An open question raised by the finding of mirror neurons in the motor cortex is that of agency discrimination. If the motor cortex is active both during execution and during passive perception of actions, how is the correct source of the action (self/other) determined? One possibility is differential activity of mirror neurons during execution and perception. Indeed single unit studies in monkeys and humans have demonstrated the existence of neurons showing increased firing rates during execution and decreased firing rates during observation of actions [43] , [44] . A possible mechanism supported by the current findings is that the problem of determining the source of sensory consequences might be partially resolved by differential responses in the sensory cortex. Our decoding results based on the activity in the auditory cortex demonstrate high classification performance of which hand was used to evoke the sound (right/left). Interestingly, we could not decode hand identity in the active condition based on the activity from frontal ROIs. This might suggest that during voluntary actions, the motor cortex modulates frontal regions regardless of effector used, and in the sensory cortex this modulation is more effector-specific. In addition to the enhanced responses to self-generated versus externally generated sounds in the auditory cortex, regions in the frontal lobe (SFG and MFG) exhibited attenuated responses during the active condition. These anatomical regions and activation patterns are compatible with brain regions associated with the default mode network [45] in which decreased activity has been shown to occur during tasks that require high executive demands (as in our fMRI active condition). Moreover, the increase in fMRI signal during the passive condition (when subjects heard their own performance) may be explained by evidence showing activation of these regions during perception of self-referenced stimuli and introspection [46] . Thus, together with sensory regions, frontal areas may play an important role in agency discrimination during action execution and perception of their sensory consequences. Previous studies have demonstrated multisensory integration of tactile information in the auditory cortex. Thus, neurons in monkey caudomedial auditory cortex and in human STG have been shown to respond to tactile stimuli [47] , [48] , [49] , [50] . Modulation of the auditory cortex by somatosensory cortex is also manifested in increased auditory sensitivity when applying tactile and auditory stimuli simultaneously [51] . Moreover, this modulation is reciprocal—TMS stimulation of the human auditory cortex has been shown to modulate temporal discrimination ability of tactile stimuli [52] . While our functional connectivity analysis supports an important role of the motor cortex in the modulation of activity in auditory cortex, in our current design we could not decouple the motor and tactile components (pressing the digital piano keys) that exists during active playing. It should be noted that in our control digit-typing task (which had similar motor and tactile components but visual instead of auditory feedback) we found activity that was not significantly different than zero in our STG ROIs. This is in better agreement with the interpretation of a predominant motor source of STG modulation, although this deserves further investigation. An ecological explanation that has been suggested for the behavioural phenomenon of sensory attenuation to self-generated sounds is that it is beneficial in avoiding desensitization of the sensory apparatus and allows increased sensitivity to external input that might have higher ecological relevance. However, under certain conditions, sensory enhancement to self-generated stimulation might be more advantageous for improved task performance. For example, reaching one's pocket in search of the car keys, it would be beneficial to increase sensitivity in auditory and somatosensory cortices. It should be noted that in our behavioural study we used 1-kHz pure tones; therefore, it remains to be seen whether these results generalize to other frequencies. In addition, different subjects participated in the behavioural and fMRI studies. Although our fMRI and behavioural results are compatible, they could nonetheless represent different underlying neural mechanisms. To conclude, our results support a model in which voluntary actions engage neural activity in the motor cortex that is stronger in the hemisphere contralateral to the active hand. We postulate that the active motor cortex sends efference copies to both ipsi and contralateral auditory cortices resulting in enhanced activity in these regions that improves sensory processing. Since anatomical and functional connections between motor and auditory cortices residing within the same hemisphere are stronger than the connections across hemispheres, this enhancement is stronger in the auditory cortex contralateral to the acting hand (see Fig. 8 ). Finally, our physiological results have two behavioural correlates. First, the enhanced activity in the auditory cortex corresponds with improved binaural hearing thresholds of self-generated sounds. Second, the sensitivity of the auditory cortex to hand identity during sound generation corresponds with improved monaural hearing thresholds when the sound-triggering hand is ipsilateral to the stimulated ear. 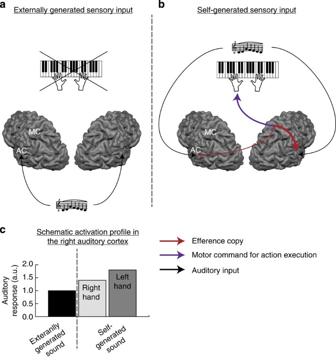Figure 8: Model of neural activity during perception of self-generated or externally generated sensory stimuli. An auditory stimulus that is generated by an external source (a) evokes similar activity in left and right auditory cortices. However, when the identical stimulus is the consequence of self-generated action (b), the activity in auditory cortices is enhanced because of excitatory efference copies (red arrows) that are sent from the active motor cortex (in the example above—right motor cortex during left hand playing). This enhancement is stronger (bold red arrow) in the auditory cortex ipsilateral, compared with the enhancement in contralateral auditory cortex (relative to the active motor cortex). The enhanced activity in STG also corresponds with increased perceptual sensitivity. (c) Model of fMRI response in right STG during unimanual left hand playing. Self-generated sound leads to enhanced activity in the auditory cortex, which is greater when the sound is generated by the left hand (andvice versafor the left STG). AC, auditory cortex; MC, motor cortex; a.u., arbitrary units. Figure 8: Model of neural activity during perception of self-generated or externally generated sensory stimuli. An auditory stimulus that is generated by an external source ( a ) evokes similar activity in left and right auditory cortices. However, when the identical stimulus is the consequence of self-generated action ( b ), the activity in auditory cortices is enhanced because of excitatory efference copies (red arrows) that are sent from the active motor cortex (in the example above—right motor cortex during left hand playing). This enhancement is stronger (bold red arrow) in the auditory cortex ipsilateral, compared with the enhancement in contralateral auditory cortex (relative to the active motor cortex). The enhanced activity in STG also corresponds with increased perceptual sensitivity. ( c ) Model of fMRI response in right STG during unimanual left hand playing. Self-generated sound leads to enhanced activity in the auditory cortex, which is greater when the sound is generated by the left hand (and vice versa for the left STG). AC, auditory cortex; MC, motor cortex; a.u., arbitrary units. Full size image fMRI study Subjects were recruited via electronic advertisements circulated among undergraduate students in the Tel-Aviv University. Every subject who met the standard inclusion criteria for participation in fMRI experiments (regardless of gender) was recruited. Thirteen healthy right-handed undergraduate students (three males; mean age 23.7, range 21–27 years) naive to the purpose of the experiment participated in this study. All subjects had normal (or corrected to normal) vision and hearing. None of them were professional musicians, although some had variant musical backgrounds. The study conformed to the guidelines and was approved by the ethical committee in the Tel-Aviv University and the Tel-Aviv Souraski Medical Center. All subjects provided written informed consent to participate in the study and were compensated for their time. The day before the experiment, subjects performed a half hour training session during which they learned to play a 7-note musical sequence on a digital piano keyboard—either with their right hand or, one octave lower, with their left hand. The next day, the subjects underwent an fMRI scan that consisted of two 5.5-min runs. Each run started and ended with a 21-s blank screen. The runs consisted of alternating experimental trials lasting 9 s and silent resting periods (9 s) in which the subjects had to fixate on a cross in the centre of the screen. During the experimental trials of the first run, the subjects had to perform the musical sequences on an MRI-compatible piano keyboard with either their right or left hands following a visual cue (‘RIGHT’/‘LEFT’; active condition) and at the practiced rate (~1.5 notes per second; active condition, Fig. 1 ). The subjects lay in a supine position during the scan with the keyboard positioned on their abdomen. Throughout the run, subjects played the musical sequence 16 times (8 with each hand) in a pseudorandomly mixed order. Performance level for each subject was calculated as % correct notes of the trained musical sequences that were played during the active condition. During the second run, the subjects looked at a fixation cross (‘+’) that changed during the experimental trials to ‘*’ to cue for the upcoming auditory stimulus. In the experimental trials they passively listened to the playback of their own performance, which was recorded during the first run (passive condition; Fig. 1 ). In the control experiment using 1-kHz tones, the subjects had to report detection of an ‘oddball’ tone of 500 Hz by pressing a button (total of four ‘oddball’ tones presented per subject; 44 correctly reported oddball tones out of 44 across all subjects). In addition, we performed an experiment in which subjects passively listened to the same 7-note musical sequences for two consecutive runs. The 7-note musical sequence was different from the one used in the main experiment. Data from these runs were used as a localizer for defining the ROI in STG (using a contrast of listen>rest). Thus, the main fMRI effects and ROI definition were independent. These data were also used to examine the order effect. The STG ROIs in the 1-kHz-tone control experiment were defined using a separate localizer run in which the subjects listened to 500 Hz tones (using a contrast of listen>rest). During the active condition of the main experimental design, the subjects played musical sequences and received online auditory feedback through MRI-compatible ‘Optoacoustics’ OPTOACTIVE headphones. Before the scans, we verified that auditory feedback through the headphones was well heard. The feedback was generated with the MIDI-OX software and each key on the digital piano keyboard was associated with one piano-like tone (arranged in the standard chromatic scale). During the passive condition, the subjects listened to the recorded playback of their own performance played by MIDI player. Thus, the auditory stimulation across conditions was identical both in timing and intensity. The rational for using musical sequences (as opposed to pure tones) was twofold: (a) to obtain high signal-to-noise ratio of evoked responses from multiple key presses (in motor cortex) and multiple sounds (in auditory cortex) and (b) to keep the experiment as ecological and engaging to the subjects as possible. Functional imaging was performed on a 3 T GE scanner with an 8-channel head coil at the Souraski Medical Center, Tel-Aviv, Israel. For each subject, 39 interleaved ascending echo-planar T2*-weighted slices were acquired for each volume, giving whole-brain coverage (slice thickness, 4 mm; slice gaps, 0 mm; in-plane resolution, 1.72 × 1.72 × 4 mm; TR, 3,000 ms; TE, 30 ms; flip angle, 90°; field of view, 220 × 220 mm 2 ; matrix size, 128 × 128). For anatomical reference, a whole-brain high-resolution T1-weighted scan (voxel size, 1 × 1 × 1 mm) was acquired for each subject. fMRI data analysis was performed using ‘Brain Voyager QX’ v. 2.3.1 software package (Brain Innovation, Maastricht, the Netherlands). Data preprocessing included cubic spline slice-time correction, trilinear/sinc three-dimensional (3D) motion correction and temporal high-pass filtering at 0.006 Hz. Both anatomical and functional images were transformed into the standardized coordinate system of Talairach [53] and data analysis was performed using the general linear model [54] . Our contrast of passive>rest resulted in regions more closely located to STG than to A1. This is in agreement with previous studies showing that primary auditory cortex (A1; Heschl Gyrus) is less sensitive to pure tones [55] . Therefore, we defined our auditory ROIs in STG ( Fig. 3a ). The general linear model was whole-brain corrected using q(FDR)<0.05, and a ROI with a maximum size of 10 mm in each axis was used. Percent signal change in each trial was defined relative to the average signal of two time points (−3 and 0; in s), with time point 0 being trial onset. The mean of three time points (3, 6 and 9 s, relative to trial onset) was taken as the representative response for each trial. Effects of interest were examined using t -tests with significance level of alpha=0.05. For visualization purposes only, the multistudy maps in Figs 2 and 3 , and in Supplementary Figs 2 and 3 were created from spatially smoothed (Gaussian filter: full-width at half-maximum=9 mm) volume–time course files of individual subjects from each experiment. To further examine the modulatory mechanisms of the motor cortex on auditory cortex, a PPI analysis [56] was performed for the active condition with right and left motor cortices as seed regions; the motor ROIs were defined by the contrast right hand>left hand and the active area around the hand knob [57] was sampled. The PPI regressors were calculated for each subject as the dot products of the z-normalized time course in the seed region of interest and the z-normalized design matrix convolved with the two-gamma haemodynamic response function. Thus, the resulting PPI design matrix for each seed region included the interactions between activity in the seed region and an experimental condition of right hand and left hands. Our PPI-based contrast (interaction of a seed region and right hand>interaction of a seed region and left hand) tested for regions that are more functionally connected with the seed region when the subjects played with one hand compared with another. Multistudy, whole-brain, PPI-based contrast was performed on spatially smoothed (Gaussian filter: full-width at half-maximum=6 mm) volume–time course files of individual subjects to identify the regions that showed the most significant beta values, indicating the strongest functional connectivity. For this analysis we collected data from additional three subjects (three females, aged 22, 24 and 25 years) and excluded data from one subject (due to completing only part of the experiment), thus leading to 15 subjects for PPI analysis. Multivoxel pattern analysis was performed to classify identity of the executing hand (right or left) under the active condition. One subject was excluded because of the lack of activation in any frontal regions, one subject was excluded because of the lack of activation in SFG and one subject was excluded because of completing only four trials in both active and passive conditions. This left 12 subjects for the decoding analysis based on fMRI signal from STG, 10 subjects for the analysis based on the signal from SFG and 11 from SFG. We used a Matlab implementation of a linear support vector machine (libsvm toolbox adopted from http://www.csie.ntu.edu.tw/~cjlin/libsvm [58] ) and performed binary classification across conditions (left versus right hand). In each iteration, two trials were left out for testing classifier accuracy (one trial out of eight from each condition) and the rest of the trials were used as the training set. As input to the classifier, we used % signal change in the sixth second relative to trial onset in each voxel from STG, MFG or SFG ROIs. For each subject, the mean performance level of the classifier across all 64 train/test data combinations was calculated. To assess statistical significance of classifier performance, a one-tailed t -test (significance level of alpha=0.05) for single sample was used on the performance level across subjects versus chance level (50%). Behavioural study The behavioural study was conducted at the Department of Communication Disorders, Tel-Aviv University, at the Sheba Medical Center, Tel Hashomer. Threshold evaluations took place in a soundproof chamber by means of a clinical GSI-61 audiometer. Stimuli were presented via TDH-39 headphones and subjects were instructed to respond by button pressing when they detected the stimulus. Binaural and monaural thresholds to air conduction 1 kHz pure tones were measured using the ‘ 1step up, 2 steps down ’ method [59] starting at 2 dBHL in 1 dB steps. If a subject did not respond in a given trial, the stimulus intensity in the following trial was increased by 1 dB; if a subject responded, the stimulus intensity in the following trial was decreased by 2 dB. The lowest intensity at which the subject reported detection in at least 50% of the presentations (with a minimum of two responses) was determined as the threshold. Subjects used one hand to trigger the auditory stimuli with a key press, when the word ‘PRESS’ appeared on a computer screen (located in front of chamber’s glass window) and the other hand to respond to the tone detection. When ‘+’ appeared on the screen, subjects looked at the experimenter press a key to trigger the auditory stimuli. Thus, differences in temporal expectation level between self and externally generated sounds were minimized [38] , [60] . In addition to the experimental paradigm, threshold evaluation at 0.5, 1, 2 and 4 kHz was performed in both ears using the ‘up-5 down-10’ clinical procedure to ascertain normal hearing thresholds (≤15 dBHL). All subjects (regardless of gender) that were recruited to the behavioural experiments had no history of hearing loss, tinnitus and ear disease and had normal (or corrected to normal) vision. Subjects provided written informed consent to participate in the study and were compensated for their time. The study conformed to the guidelines and was approved by the ethical committee of the Tel-Aviv University. Auditory stimulus consisted of a 1-kHz pure tone with a duration of 300 ms and a rise/decay time of 25 ms (constructed by means of MATLAB v.7.12 software—MathWorks). The tone was delivered by a computer connected to the audiometer. Binaural hearing thresholds Sixteen right-handed undergraduate students participated in this experiment (nine males; mean age, 24.18, range 21–31 years). Binaural thresholds were measured in the two following conditions: Active condition—in which the subjects pressed a key with their right index finger to trigger auditory stimuli. Passive condition—in which the subjects watched the experimenter press a key to trigger auditory stimuli. Threshold evaluation was performed three times with repetition order pseudorandomly mixed across conditions. For each subject, the mean threshold across the three repetitions of each condition was calculated. Binaural sensitivity and criterion estimation In order to assess sensitivity (d′) and criterion (c), 11 right-handed undergraduate students participated in the experiment. The data from one subject were excluded due to ceiling performance (no false-alarm trials) leaving 10 subjects (2 males; mean age, 24.7, range 21–31 years). First, binaural auditory thresholds were measured under the active and passive conditions (one repetition each). The lower of the two thresholds was used in the following stage, as the intensity of presented stimuli. Next, the subjects performed 10 blocks of active and 10 blocks of passive conditions (pseudorandomly mixed). Each block comprised 10 single trials. In 50% of the trials in each block, the key press triggered a sound (at the intensity determined from the first stage), whereas in the remaining 50% of trials no sound was delivered. Trial type order (sound/no-sound) was pseudorandomly mixed within the block. The subjects were instructed to report when they heard the sound. In this manner, we could measure the probability of hits and false alarms to calculate d′ and criterion (c) according to the Signal Detection Theory [61] . Monaural hearing thresholds Fourteen right-handed and one left-handed undergraduate students participated in the experiment (seven males; mean age, 24.18, range 22–27 years). For each subject, thresholds were measured in each ear (left and right), separately. Data from six ears were excluded because of technical problems (three ears) or failure to complete the experimental protocol (three ears). Thus, leaving data from 22 ears of 13 subjects. Monaural hearing thresholds were estimated in the two following conditions: Ipsilateral condition—in which the stimulated ear and the hand used to trigger the sound were on the same side (that is, left hand key presses and left ear stimulation or right hand key presses and right ear stimulation). Contralateral condition—in which the stimulated ear and the hand used to trigger the sound were on opposite sides (that is, left hand key presses and right ear stimulation or right hand key presses and left ear stimulation). Before each block, subjects were instructed with which hand to press a key in order to trigger the sound. Owing to spatial congruency between the hand pressing the key and the stimulated ear in the ipsilateral condition (that is, both were located at the left or right sides of the subject), seven subjects (10 ears) pressed the key located on the opposite side of the body (for example, subjects pressed with their left hand a key placed on the right side of the keyboard and vice versa for the right hand). In this manner, the hand in the ipsilateral condition was in the opposite hemispace of the stimulated ear. Each condition (ipsi/contra), for each ear, was repeated twice; condition order was pseudorandomized. If monaural threshold measurements were completed within 20 min, additional repetitions for each condition were added, in mixed order. Thus, for eight subjects (12 ears) each condition was repeated twice and for five subjects (10 ears) each condition was repeated three times. For each subject, the mean monaural threshold across all available repetitions in each condition was calculated. How to cite this article : Reznik, D. et al . Lateralized enhancement of auditory cortex activity and increased sensitivity to self-generated sounds. Nat. Commun. 5:4059 doi: 10.1038/ncomms5059 (2014).